Unfavourable environment limits social conflict inYuhina brunneiceps Identifying the factors that modulate cooperative and competitive behaviours is the key to understanding social evolution. However, how ecological factors affect social conflict and their fitness consequences remain relatively unexplored. Here, using both a game-theoretical model and empirical data, we show that Taiwan yuhinas ( Yuhina brunneiceps )—a joint-nesting species in which group members are unrelated—employ more cooperative strategies in unfavourable environmental conditions. Fighting duration was lower, fewer total eggs were laid and incubation was more likely to start after all females completed egg laying (which causes more synchronous egg hatching). Surprisingly, as a consequence, there were more surviving offspring in unfavourable conditions because the cooperative strategies resulted in fewer dead nestlings. To our knowledge, this study is the first theoretical analysis and empirical study demonstrating that an unfavourable environment reduces social conflict and results in better fitness consequences in social vertebrates. Cooperation and conflict are inevitable and opposing forces within social groups [1] , [2] , [3] , [4] . Much attention has focused on how ecological factors affect the benefits of cooperation [5] . For example, lower predation risk, greater foraging efficiency and better access to critical resources have been considered the three general classes of social benefits favouring group living [6] . It is also well accepted that ecological factors have a critical role in the evolution of social groups, such as ecological constraints [7] and fluctuating environments [8] , [9] that favour group formation and cooperative breeding. However, social conflict and its resolution within a stable social group have mostly been understood by studying intrinsic individual properties, such as genetic relatedness between interacting individuals [10] , resource holding power [11] , and behavioural strategies such as tit-for-tat responding [12] , punishment [13] and policing [14] , [15] . Although the cost c and benefit b terms in Hamilton's rule (rb-c>0) inherently involve ecology, the precise role of ecology in influencing within-group conflict remains poorly understood [16] , [17] , presumably because the relative importance of social and ecological factors are often difficult to disentangle in most social animals forming groups with kin. In plural breeding species, where two or more females breed in a social group and provide parental care to their offspring, conflict over the relative share of reproduction is often intense. Extreme expressions of social conflict, such as egg destruction and infanticide, commonly occur in many plural breeding birds, mammals and social hymenoptera, for example refs 18 , 19 , 20 . Plural breeding species are therefore good subjects for studying how group members resolve breeding conflicts. However, little is known about how ecological factors affect the intensity and the fitness consequences of these social conflicts. We develop a game-theoretical model to explore the theoretical consequences of how ecological factors affect social conflict in the context of cooperatively breeding species. We make four general assumptions to depict the tragedy of the common scenario in the joint-nesting system of yuhinas: first, we assume that offspring fitness increases as its share of group resources increases; second, an offspring's share of group resources decreases as joint-brood size increases, and increases as its parent's competitive effort increases; third, breeding adults sustain personal costs of producing young and competing for group resources in the form of reduced future fitness; and finally, we assume that ecological conditions influence the costs of investing in offspring production and engaging in social conflict, and these costs are higher in poorer ecological conditions. We then studied how ecological conditions affect social conflict and fitness of plural breeding and joint-nesting Taiwan yuhinas ( Y. brunneiceps ) to test the predictions of our models ( Fig. 1 ). Most individuals (about 90%) live in social groups that are comprised of two to three unrelated monogamous pairs and sometimes one non-breeding helper [21] . The joint-nesting behaviour of yuhinas, in which multiple females contribute eggs to a group nest and provide parental care, is a rare form of cooperative breeding [22] . We examined four types of competitive strategies between co-breeding female yuhinas, namely, preventing other co-breeding females' access to the nest during egg laying; laying more eggs; early onset of nocturnal incubation to facilitate the earlier development of one's own eggs; and egg tossing. 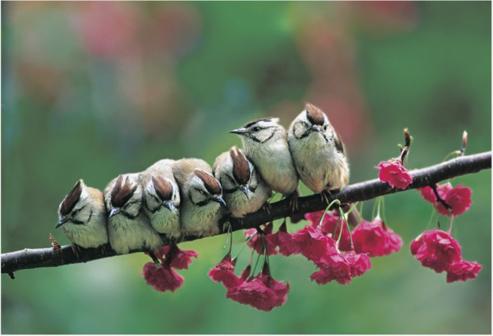Figure 1: A group of Taiwan yuhinas huddled together. (© I.-D. Lin). Figure 1: A group of Taiwan yuhinas huddled together. (© I.-D. Lin). Full size image Description of the cooperatively breeding model We explore the theoretical consequences of how ecological factors affect social conflict in the context of cooperatively breeding species. We explicitly consider that ecology can affect the costs of offspring production and cost of investing in social conflict in groups with n breeders. We assume that if ecological conditions are poor, the cost of producing offspring is higher. Specifically, building on the costly young model [23] , [24] , [25] , we assume that an individual young's fitness, s ( f , x ), declines linearly with total brood size, f+(n −1 )f ′, where a focal individual produces f offspring and f ′ represents the population average number of a non-focal individual's offspring production. We also assume that parents' competitive effort, x , also influences the offspring's share of group resources and thus offspring fitness. For example, adult females' competitive effort for early egg laying and early onset of nocturnal incubation resulted in asynchronous hatching, and early hatchlings had a competitive advantage in joint-nesting yuhinas (see text for details). An individual young's fitness is where x ′ represents the average population competitive effort, offspring's fitness is proportional to their parents' competitive effort and a represents the rate of decline of offspring fitness with the increase in total brood size ( a > n ( f +( n −1) f ′) so that offspring fitness s will be greater than zero). Small values of a indicate that there is a larger negative impact on offspring fitness with larger brood size. We also assume that producing offspring and investing in competitive effort entail personal costs, e f f and e x x , respectively; e f and e x increase as ecological conditions deteriorate. Furthermore, we assume that investing in current reproduction and social conflict entails an accelerating future fitness cost [26] to the mothers and thus the cost function is equal to ( e f f+e x x ) [2] . To determine the evolutionarily stable producing and competing strategies, we adopt the 'direct fitness' approach [27] , [28] , [29] ; this is equivalent to the neighbour-modulated fitness of Hamilton [12] . The direct fitness payoff of a group member is given by The evolutionarily stable levels of competitive effort x ′ and number of offspring produced f* adopted by group members must then satisfy where r denotes the relatedness among group members. This equation represents the condition that the evolutionarily stable levels of competitive effect and brood size should be the ones yielding the highest fitness in a population of individuals exhibiting those same strategies. Therefore, no alternative mutant strategy can invade the population. The solutions, which correspond to the maximum of the individual fitness, are equal to where . Results of the cooperatively breeding model As yuhina group members are almost all unrelated to each other, we present the results of the model for non-kin groups ( r =0; results for related groups are qualitatively the same). As can be verified by checking the derivatives of x* and f* with respect to each of the contained variables, group members' competitive effort, x* , decreases as the cost of investing in competitive effort, e x , increases, the cost of investing in offspring production, e f , increases, and sensitivity of offspring fitness to brood size, a , increases ( Supplementary Fig. S1a ). In other words, not surprisingly, if poor ecological conditions increase the personal cost of competing (larger e x ), social conflict will be lower. Interestingly, social conflict will also be lower if an unfavourable environment increases the cost of producing young (larger e f ). This is because if the cost of producing young is higher, individuals will invest less in current reproduction and thus reduce the investment in competition, even if ecological conditions do not influence the personal cost of competitive effort directly. This result is true whether the costs of investing in offspring production and social conflict increase linearly or nonlinearly (that is, whether the exponent of the cost function is equal to or greater than one) in most of the biologically realistic parameter space (that is, e f <1 and n >1). It is also intriguing to see that social conflict decreases as poor ecological conditions increase the difficulty of rearing young (smaller a ). In this case, poor ecological conditions lower offspring fitness, which leads to individuals investing less in competing for current reproduction. The number of offspring produced, f* , decreases as the cost of investing in offspring production, e f , increases, decreases slightly as sensitivity of offspring fitness to brood size, 1/ a , increases ( Supplementary Fig. S1b ), but is not affected by the cost of investing in competitive effort, e x . Counterintuitively, the offspring fitness, s[f , f ′, x , x ′], increases ( Supplementary Fig. S1c ), but total surviving offspring, n f* s[f, f ′, x, x ′], can decrease or increase as ecological conditions become worse if ecology affects the cost of producing young ( Supplementary Fig. S1d ). This occurs because when poor ecological conditions lead to a higher cost of investing in offspring production, the number of offspring produced is lower; offspring share the group's resources with fewer broodmates, which leads to higher offspring survival. If poor ecological conditions mainly affect the sensitivity of offspring to brood size, offspring survival will be lower in such a scenario ( Supplementary Fig. S1c ). Description and results of the general model Building on the influential framework of Frank [17] , see also ref. 30 , we focus on how ecology affects the tension between group productivity and individual competition for a share of group productivity. The fitness of an individual in a group, w ij , is: where z ij and c ( z ij , E ) are competitive effort and the personal cost of the competitive effort, respectively, of the j th individual of the i th group. E indicates ecological condition (larger E represents better ecological conditions). z i is the average level of competitive effort and g ( z i , E ) is the group productivity function in the i th group. Frank and subsequent models [17] , [27] , [31] have focused on specific group productivity functions and no personal cost of social conflict. Here, we explore a range of alternative possibilities, subject only to the conditions that: (a) ∂ g /∂ z <0 and ∂ 2 g /∂ z 2 ≤0, representing group productivity as a decreasing and linear or accelerating function of competitive effort; and (b) ∂ 2 g /∂ z ∂ E >0 and ∂ g /∂ E ≥0, indicating that group productivity is an increasing function of ecological condition with diminishing returns but group productivity decreases less rapidly in good ecological conditions; (c) ∂ c /∂ z >0, ∂ 2 c /∂ z 2 >0 and ∂ 2 c /∂ z ∂ E <0, implying that proportional personal cost is an increasing and accelerating function of competitive effort [26] , but that this cost increases less rapidly in good ecological conditions. Using the direct fitness approach (or neighbour-modulated fitness) [27] , [28] , the evolutionarily stable level of competitive effort z * must satisfy where r is the relatedness between group members. As the above equation holds for all values of E and z , we can differentiate with respect to E to obtain, after some rearrangement, which, given the assumptions stated above (∂ g /∂ z <0, ∂ 2 g /∂ z 2 ≤0, ∂ 2 g/ ∂ z ∂ E >0, ∂ g/ ∂ E ≥0, ∂ c /∂ z >0, ∂ 2 c /∂ z 2 >0 and ∂ 2 c /∂ z ∂ E <0), must be positive. Thus, social conflict is predicted to be lower in unfavourable ecological conditions, regardless of the precise form of the various cost and benefit functions. When group productivity is mainly determined by social conflict, that is, ∂ g /∂ E =0, group members compete for a fixed amount of resources, which is not affected by ecological conditions. In this scenario, group productivity is predicted to be higher in unfavourable environments because social conflict is less. However, when ecological conditions influence both group benefits and social conflict, the effects of ecology on group productivity cannot be determined without the specific information of how ecology affects the group benefits and social conflict (that is, both g ( z i , E ) and c ( z ij , E ) functions need to be explicit). Competitive strategies in yuhinas We discovered that female group members often aggressively competed for access to the nest during egg laying with tussling behaviours ( Supplementary Movie 1 ). All the tussling events and egg-laying attempts occurred early in the morning, usually within 5 min of hearing the first male yuhina songs. Tussling behaviour occurred in almost all nests (97%, n =35/36) in which more than one female laid eggs on the same day. Longer tussling duration was associated with more females successfully laying eggs (generalized linear mixed model (GLMM), F 1,44 =56.32, P <0.001, while controlling for the effect of laying day). Nevertheless, we documented 24 cases out of 61 tussling events (39%) in which one female prevented other females from laying by tussling. Tussling events were more likely to occur when the benefit of laying eggs was higher, that is, before nocturnal incubation started (86%, 49/57 cases, compared with 43%, 12/28 cases on the days after nocturnal incubation started, Fisher exact test, P <0.01). This benefit arises because eggs laid before the onset of nocturnal incubation are more likely to hatch earlier ( Supplementary Fig. S2 ). These observations together demonstrate that tussling is an important competitive strategy affecting contributions to the communal clutch in yuhinas. In addition to direct physical aggression, the number of offspring produced is also an important competitive strategy. In yuhinas, offspring body weight decreased (GLMM, slope=−0.71±0.21, F 1,95 =11.71, P <0.001) and both the absolute number and proportion of offspring that died increased as joint-brood size increased (GLMM, slope=0.17±0.06, F 1,11 =6.97, P <0.01; proportion: slope=0.12±0.05, F 1,11 =5.93, P <0.05). Thus, laying more eggs increases an individual's personal share of group resources but can drive the joint-clutch size larger than the most productive size (see also ref. 32 ). Early onset of nocturnal incubation is a third important competitive strategy because eggs laid after incubation onset hatch later and those chicks are at a competitive disadvantage. The number of eggs hatching on the first day significantly increased with the number of eggs incubated on the first day of nocturnal incubation ( Supplementary Fig. S2 , Spearman rank test, r =0.475, P <0.01, n =37 nests). Thus, asynchronous hatching was associated with the early onset of nocturnal incubation. Egg tossing is a fourth possible competitive strategy, but it occurred only rarely in 8.3% (3/36) of nests. In all three cases, eggs were removed immediately after tussling behaviours ended. To further test the role of egg tossing in egg-laying conflict, we conducted model egg addition experiments in nine nests. In six of these nests, a model egg was added before egg laying started. In two cases, these eggs were buried under the nesting materials, and in four cases, these eggs were accepted and incubated until the end of the incubation period. Likewise, no egg tossing occurred in the three cases where a model egg was added on the second day of egg laying. This evidence indicates that egg tossing is not an important competitive strategy for yuhinas. Our results suggest that the first three competitive strategies of female yuhinas—tussling, laying more eggs and onset of nocturnal incubation—are interconnected strategies. Females that successfully competed for laying more eggs in the first 2 days of the egg-laying period were also more likely to start nocturnal incubation. In 19/22 nests, the female that laid more eggs in the first 2 days also initiated the nocturnal incubation. This female was the alpha female in 11 cases, beta female in 7 cases and gamma female in 1 case. Early onset of nocturnal incubation thus ensures that the females that successfully competed to lay more eggs also have earlier-hatching eggs. Early-hatching nestlings had a competitive provisioning advantage; they obtained food at shorter time intervals ( Fig. 2a , GLMM, F 1,1098 =5.61, P =0.02) and were heavier than the late-hatching nestlings in the asynchronously hatching nests ( Fig. 2b , GLMM, F 1,25 =7.54, P <0.01). Although the number of eggs laid and onset of incubation do not involve direct physical aggression, both are important competitive strategies, together with tussling, in the joint-nesting system of yuhinas (summarized in Supplementary Fig. S3 ). 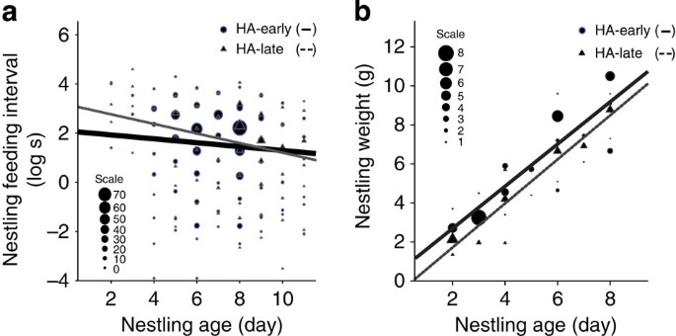Figure 2: The effect of hatching order on offspring fitness components. The relationship between hatching order (early hatching or late hatching) in asynchronously hatching nests and (a) the nestling feeding interval (intervals between two feeding events for a nestling) and (b) nestling weight at different ages. Figure 2: The effect of hatching order on offspring fitness components. The relationship between hatching order (early hatching or late hatching) in asynchronously hatching nests and ( a ) the nestling feeding interval (intervals between two feeding events for a nestling) and ( b ) nestling weight at different ages. Full size image Ecology and social conflicts in yuhinas We next investigated how ecology influences social conflict and fitness in co-breeding female yuhinas. In our high-altitude and sub-tropical montane cloud forest study site, high rainfall represented an unfavourable ecological condition for the birds. Overcast, foggy, and rainy weather often prevailed for many hours. We used 5-mm average daily rainfall as the cutoff point for good versus poor weather conditions (see Supporting Information ). In the high-rainfall condition (daily average >5 mm), it rained for prolonged periods (9.26±0.5 h per day, n =161 days), compared with the low-rainfall condition (2.05±0.11 h, n =146 days) (two-sample t -test, t 179 =14.59, P <0.001). High rainfall thus forces the birds to perform most of their daily activities in the rain. We indeed found evidence of negative influences of high rainfall: adult foraging efficiency (measured as nestling provisioning rate) significantly decreased with increasing rainfall (GLMM, F 1,288 =23.4, P <0.001); and fewer nests were initiated on rainy days (45.2%, 181/330 nests initiated in days with 3-day average daily rainfall >5 mm compared with 53.3%, 193/362 days with 3-day average daily rainfall <5 mm; λ =4.6, P =0.03). Both results imply that high rainfall represents a poor environmental condition for breeding (see also refs 33 , 34 ). Other studies have also documented a negative effect of heavy rainfall for small birds like yuhinas (12 g) for two compounding reasons. First, it is energetically costly for animals to thermoregulate and perform foraging and agonistic activities in the rain (for example, ref. 35 ). This cost occurs because surface water conducts heat away from an animal 20–30 times faster than in dry air, a problem that is especially significant for small birds because of their large surface area to volume ratios. Second, it is also well established that rainfall reduces insect activity (see ref. 36 for an example in a similar ecosystem), making foraging more difficult for insectivores. It might be thought that more rainfall would increase biomass production and thus have a positive effect on subsequent provisioning of young. However, this is not the case for yuhinas: nestlings from nests initiated during high- versus low-rainfall periods on average received similar numbers of provisioned items (GLMM, F 1,91 =0.74, P =0.39) and of similar prey sizes (GLMM, F 1,26 =0.65, P =0.42). Furthermore, the 3-day average rainfall during the egg-laying period was not correlated with the rainfall in the nestling period 2–3 weeks later (Spearman rank test, P =0.345, n =30). Thus, more rainfall during the egg-laying period did not result in a better or worse environment for provisioning young in yuhinas. We used average rainfall in the 3 days before nocturnal incubation commences to represent the ecological condition because this is the period in which all three competitive strategies (tussling, egg laying and onset of nocturnal incubation) occurred. As predicted by our model, we found that co-breeding females competed less intensely when ecological conditions were poor, that is, higher rainfall. We distinguished two types of tussling behaviours, escalated and non-escalated. A mixed model analysis showed that the duration of escalated tussling events was significantly influenced by its timing relative to incubation (days before versus after the start of nocturnal incubation) ( Fig. 3a , GLMM, F 3,43 =44.25, P <0.001) and by the rainfall ( Fig. 3b , F 1,27 =5.03, P =0.02) but not by the group size ( F 1,27 =0.30, P =0.58). Escalated tussling events rarely occurred after nocturnal incubation started. The duration of non-escalated tussling behaviours was not affected by timing relative to nocturnal incubation or rainfall (GLMM, F 1,30 =0.74, P =0.39). 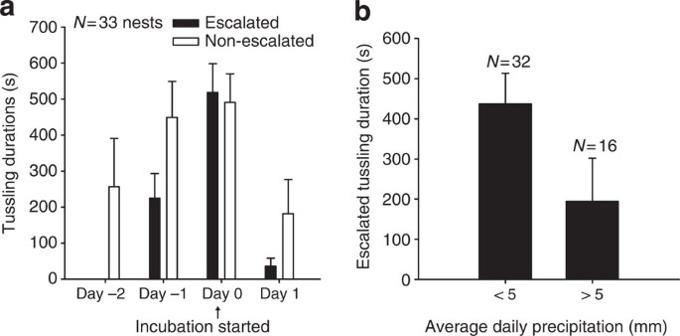Figure 3: The effect of timing and rainfall on female tussling durations. Tussling duration in relation to (a) the days relative to the onset of nocturnal incubation and (b) average daily rainfall before the onset of nocturnal incubation (sample size represents number of tussling events). Day 0 represents the day nocturnal incubation starts, in which females lay eggs in the early morning and the nocturnal incubator starts incubating eggs that same evening. Day −1 indicates 1 day before the day nocturnal incubation starts. Error bars represent s.e. Figure 3: The effect of timing and rainfall on female tussling durations. Tussling duration in relation to ( a ) the days relative to the onset of nocturnal incubation and ( b ) average daily rainfall before the onset of nocturnal incubation (sample size represents number of tussling events). Day 0 represents the day nocturnal incubation starts, in which females lay eggs in the early morning and the nocturnal incubator starts incubating eggs that same evening. Day −1 indicates 1 day before the day nocturnal incubation starts. Error bars represent s.e. Full size image Rainfall had a significant effect on the number of eggs produced and offspring quality. As predicted, more eggs were produced during periods of favourable ecological conditions (low rainfall). However, the number of total surviving offspring (representing group productivity) was lower in nests initiated during favourable ecological conditions than those initiated during poor conditions ( Fig. 4a , GLMM, the interaction effect between rainfall and nestling age, F 1,66 =4.72, P <0.05, controlling for the effect of number of females). The day (relative to the first egg-laying day) of the onset of nocturnal incubation was not affected by rainfall (GLMM, F 1,32 =0.8, P =0.379). As a consequence, when there was less rain (rainfall <5 mm), eggs were more likely to be added to a clutch after incubation had started, compared with nests active when there was more rain (rainfall >5 mm, Fig. 4b , Fisher exact test, P <0.01). Therefore, hatching was significantly more likely to be asynchronous when there was less rain (67%, 14/21 nests) versus when there was more rain (18%, 2/11 nests, Fisher exact test, P =0.02). Also as predicted, nestling condition was better in nests with eggs laid during poor ecological conditions. Counterintuitively but predicted by our model, nestlings grew significantly faster and heavier in these nests ( Fig. 4c , GLMM, the interaction effect between rainfall and nestling age, F 1,94 =17.51, P <0.001). As a consequence, late-hatching nestlings were more likely to die in nests with eggs laid during favourable conditions within groups of a cooperative species ( Fig. 4c,d , Fisher exact test, P =0.012). The 'tragedy of the commons' [37] scenario, whereby individuals compete for a higher share of group resources at the cost of group productivity, was thus avoided during unfavourable conditions in yuhinas. 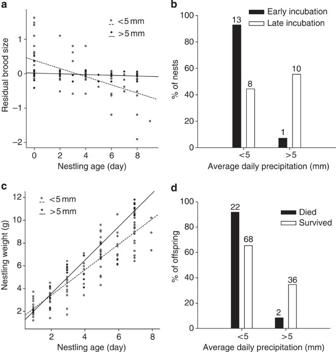Figure 4: Consequences of rainfall level on yuhina breeding. (a) The relationship between rainfall and residual joint-brood size. Day 0 represents number of eggs. (b) The relationship between rainfall and the occurrence of different onsets of nocturnal incubation. (c) The relationship between rainfall and nestling weight. (d) The fates of offspring in relation to average daily rainfall before the onset of nocturnal incubation. 'Survived' nestlings were successfully fledging nestlings. Numbers above each bar indicate sample sizes. Figure 4: Consequences of rainfall level on yuhina breeding. ( a ) The relationship between rainfall and residual joint-brood size. Day 0 represents number of eggs. ( b ) The relationship between rainfall and the occurrence of different onsets of nocturnal incubation. ( c ) The relationship between rainfall and nestling weight. ( d ) The fates of offspring in relation to average daily rainfall before the onset of nocturnal incubation. 'Survived' nestlings were successfully fledging nestlings. Numbers above each bar indicate sample sizes. Full size image Repression of competition has been proposed to be a major force shaping the evolution of cooperation because if group members cannot compete, each individual can only increase its own success by increasing the efficiency and productivity of the whole group [38] . However, there are relatively few empirical studies on how ecology influences social conflict (see refs 6 , 39 ) and the fitness consequences associated with the conflict. One exception is from non-cooperatively breeding olive baboons, in which aggressive interactions between dominants and subordinates were found to decrease in the 1984 East African drought [40] . This reduction of social conflict occurred because baboons had to devote their entire day to foraging in this poor ecological context, as the grassland biomass was severely reduced. Thus, this study provides preliminary support for our model's prediction that a higher personal cost of social aggression in unfavourable ecological conditions limits social conflict. The idea that poor ecological conditions can limit social conflict and counterintuitively lead to a better outcome was proposed by the great ancient Chinese military strategist, Sun Tzu, 2,500 years ago. Our paper provides the first game-theoretical model and biological example supporting the idea that unfavourable ecological conditions can limit the within-group conflict and prevent the tragedy of the commons. This result stands in contrast to several recent studies in which social conflict was more intense in poor ecological conditions [41] , [42] , [43] . We believe that the key difference is that in our specific case and general model, group resources or benefits of cooperation are important for improving individual fitness, where in these other cases, ecological condition is the main determinant of group resources, and cooperation does not increase group productivity. Thus, individuals invest more to compete for personal gain in unfavourable environments. The general understanding of how ecology influences cooperation and social conflict remains largely unexplored, and more studies are clearly needed. The study species Yuhinas are effectively obligatory cooperative breeders. Not only is the proportion of solitary breeders very small (only 14% (22/161) of group-years involved solitary breeders, and only 12% (38/318) of nests were built by solitary breeders in our long-term study), but more importantly, these solitary breeding pairs have extremely low breeding success (S.-F. Shen, unpublished data). Our data showed that the benefits of group breeding in yuhinas are associated with strategies of coping with an unpredictable environment, caused by high predation risk and severe weather (for example, heavy rain and typhoons) [21] , [44] . Yuhinas reduced their workload during incubation and nestling provisioning when breeding in larger groups [45] . Adult survival rate was higher in larger groups. Larger groups also re-nested faster after nest failures and had more nesting attempts (up to nine total nesting attempts and three successful attempts) in a season. However, as per capita offspring production decreased as group size increased, two-pair groups had highest lifetime reproductive success and represented the most common group size in our population (S.-F. Shen, unpublished data). We therefore believe it is reasonable to exclude solitary breeding as an 'outside option' in our analyses, and focus on within-group conflict in joint-nesting groups. Field and lab methods The detailed behavioural data analyzed in this study were collected during the 2004 through 2007 breeding seasons. In each year, we closely monitored 17, 15, 14 and 19 breeding groups, respectively. This study was conducted at the National Taiwan University Highlands Experiment Farm at Meifeng, in the mountains of central Taiwan (24 05′N, 121 10′E, elevation 2,150 m) [21] . The linear dominance hierarchy of each gender was determined by the patterns of displacement and chasing [21] . Higher-ranked individuals consistently chased and displaced lower-ranked, same-gender members of the group. The relative reproductive share between dominants and subordinates varied but was typically low in a given nesting attempt (with average reproductive skew=0.19) [21] , and reproductive share also varied among different nesting attempts within a season (S.-F. Shen, unpublished data). Therefore, joint-brood size and per capita brood size are good approximations of individual fitness. To observe egg laying, nocturnal incubators, physical interaction behaviours of known individuals at the nest and group provisioning behaviour, we implanted RFID transponders (Trovan) under the skin of adult birds for remote monitoring of individual nest visits. The circular antenna for the transponders was mounted under the nest. A bullet camera (1/3″ B/W IR, Yaba) was mounted above each nest and recording was continuous from 0400 to 2000 hours every day to cover the whole range of adult and nestling activities. Onset of nocturnal incubation (that is, eggs were incubated in the evening and thereafter adults incubated eggs continuously), egg-tossing events, egg-hatching patterns, group provisioning behaviour and nestling survival were monitored by this recording system. The distribution of provisioned food among nestlings and food size were also recorded by the video system. We use non-toxic acrylic paint to mark the head and bill of nestlings for nestling identification. We sex typed individuals with 2550F and 2718R primers [46] . Each individual was genotyped at 6–9 microsatellite loci for kinship assignment [21] . The primer sequences are GC-GATA 8, GC-GATA11, GC-GATA13, GA-GATA 15 and GC-GATA 22 [47] ; lsgata 07 and lsgata 17 [48] ; T39 [49] ; and 1311 was an unpublished primer pair (S.-H. Li, unpublished data). Data sampling We fully recorded 37 nests during the incubation and nestling periods. We successfully recorded 85 days of egg-laying behaviour from 36 nests; 61 tussling events were observed in these recordings. Owing to recording timing and quality, we were able to quantify tussling duration in only 33 nests. Rainfall data are missing for one nest, yielding 32 nests with tussling duration and rainfall data. The group size of egg-laying-monitored nests ranged from three to six adults. We did not obtain tussling data from every group we monitored. Data from 34 nests with a total of 288 h of recording were used to analyze the group's nestling provisioning behaviour. Rainfall in this analysis represents hourly averages. Rainfall data were collected by an automatic weather station located in the study site and operated by the Mei-Feng Highland Experimental Farm of National Taiwan University. We observed that two females often visited the nest at the same time and engaged in physical interactions, a behaviour we call tussling. Two types of tussling behaviour were distinguished based on the severity of the behaviour. Escalated tussling behaviour was noted if the female on top tried to push or peck the other female sitting on the nest, whereas non-escalated tussling behaviour was scored if one female simply stood on the other female. The two types of tussling behaviour are qualitatively different levels of agonistic behaviour between females at the nest—physically aggressive pushing and pecking versus non-aggressive standing. The former is a very costly behaviour, the latter is not, so we divided 'tussling' into two levels and examined the effects of rainfall on the rate of each type of tussling. We also distinguished two levels of hatching synchrony, obtained by our video recording system, with synchronous hatching occurring when all nestlings hatched within 12 h and asynchronous hatching occurring when nestlings hatched over a period greater than 12 h. We conducted model egg addition experiments in nine nests to assess the ability of yuhinas to distinguish their own eggs from foreign eggs. The model eggs were real yuhina eggs with the contents blown out and replaced by wall-patch putty; some staples were added to match the weight of a real yuhina egg and to ensure that they rolled normally. We used the average daily rainfall 3 days before the onset of nocturnal incubation (incubation of eggs through the night) as an indication of ecological conditions during laying. Nocturnal incubation is critical for egg development, and once it started, group members continuously incubated the eggs day and night. The nesting and rainfall data analyzed in this study were collected during the 1997, 1998, 2000 and 2003–2007 breeding seasons. We found a total of 330 nests with associated rainfall data. We used 5-mm average daily rainfall before the onset of nocturnal incubation as the cutoff point of weather condition because about half (181/330 nests) of the nests were initiated in days with average rainfall <5 mm. Of these 8 years' worth of rainfall and nesting data, we only had the provisioning and tussling data from the transponder and video recording systems in the last 4 years. Statistical analysis We used a GLMM to analyze nestling weight, number of surviving offspring, brood size, group provisioning behaviour and variation in duration of escalated and non-escalated tussling events, including nestling ID (for the nestling weight analysis) and group identity (for all analyses) as random factor(s) to account for a possible correlation of behaviours between individuals of the same group. How to cite this article: Shen, S.-F. et al . Unfavourable environment limits social conflict in Yuhina brunneiceps . Nat. Commun. 3:885 doi: 10.1038/ncomms1894 (2012).